Impact-induced shock and the formation of natural quasicrystals in the early solar system The discovery of a natural quasicrystal, icosahedrite (Al 63 Cu 24 Fe 13 ), accompanied by khatyrkite (CuAl 2 ) and cupalite (CuAl) in the CV3 carbonaceous chondrite Khatyrka has posed a mystery as to what extraterrestrial processes led to the formation and preservation of these metal alloys. Here we present a range of evidence, including the discovery of high-pressure phases never observed before in a CV3 chondrite, indicating that an impact shock generated a heterogeneous distribution of pressures and temperatures in which some portions reached at least 5 GPa and 1,200 °C. The conditions were sufficient to melt Al–Cu-bearing minerals, which then rapidly solidified into icosahedrite and other Al–Cu metal phases. The meteorite also contains heretofore unobserved phases of iron–nickel and iron sulphide with substantial amounts of Al and Cu. The presence of these phases in Khatyrka provides further proof that the Al–Cu alloys are natural products of unusual processes that occurred in the early solar system. Icosahedrite (Al 63 Cu 24 Fe 13 ) [1] , [2] , an alloy displaying a three-dimensional icosahedral symmetry strictly forbidden for crystals [3] , [4] , represents the first and, to date, the only known naturally occurring quasicrystal. It was discovered in the Khatyrka meteorite [5] , [6] , [7] , an oxidized subgroup (Allende-like) CV3 carbonaceous chondrite (CV3 CC) that formed at least 4.5 billion years ago. The preservation of a quasicrystal in a meteorite that formed at the early stages of the solar system indicates that it can be stable over cosmic time scales, giving new insights on the existence and stability of these materials in nature [5] , [6] . However, the processes that produced this unusual assemblage have been a mystery, as the highly reducing conditions implied by the presence of metallic Al are unknown for natural terrestrial materials and, before our studies, for meteorites. Moreover, the combination of metallic Al (high temperature refractory lithophile) with metallic Cu (low temperature chalcophile) is totally unexpected. The results presented in this paper attempt to address these issues through a petrological investigation of sample no. 125 of the Khatyrka meteorite, a sample that provides clear evidence that the meteorite was subjected to a high-pressure impact shock, supplemented by studies of individual phases found in sample nos: 5, 121 and 126 (ref. 7 ). On the basis of the new data, our hypothesis is that the shock produced a heterogeneous distribution of high pressure and temperature, with localized melting of Al–Cu-bearing minerals followed by rapid cooling. We discuss two plausible scenarios for how the alloys initially formed that are consistent with the observations: shock-induced melting of Al–Cu-bearing iron–nickel and iron sulphide, or solar nebula origin followed later by shock melting and rapid cooling of Al–Cu-bearing minerals. Description of samples Sample no. 125 is part of the same CV3 CC as nos: 5 and 121 (ref. 7 ). The correlation is based on O-isotope measurements of an olivine grain ( Fig. 1 ), and the presence of the same types of minerals and rare Cu–Al phases found in the other Khatyrka samples [5] , [6] , [7] . Also, the shocked portion of no. 125 has the appearance of a compressed (as from shock) CV3 matrix ( Fig. 2b ). Figure 3 shows a side-by-side comparison of the compressed matrix in no. 125 and uncompressed matrix in no. 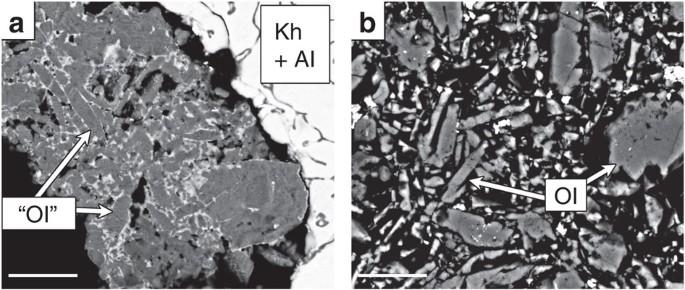Figure 3: Comparison of shocked and unshocked textures. Backscattered electron images of the shocked silicate textures in grain no. 125 (a) compared with the unshocked textures in Khatyrka matrix (b) from grain no. 5. Note that the ‘olivine’ grains in the left image have the same sizes and distinctive shapes as those in unshocked Khatyrka matrix, showing that the matrix was the precursor for the shocked silicates. Al, metallic aluminium; Kh, khatyrkite; Ol, olivine; ‘Ol’, shocked olivine grains, now consisting of ahrensite+forsterite+glass+spinels. Scale bars, 10 μm. 121 (ref. 7 ). Because all of the grains in this meteorite are so small, we only have polished grain mounts and not thin sections. Thus, we cannot apply the usual shock estimates based on optical properties such as those introduced by Stöffler et al. [8] and Scott et al. [9] (for example, undulatory extinctions and planar fractures in olivine). Figure 3 clearly shows that the matrix of the unshocked grain no. 5 is very uncompacted (unlike, for example, Leoville, a reduced-subgroup CV3 with a highly compacted and lineated fabric). However, two of the grains of Khatyrka contain the high-pressure phases ahrensite [10] (Fe-rich ringwoodite) and stishovite, and it is from these that we derive the shock history of this meteorite. We note that shock effects in meteorites can be highly localized and difficult to identify; hence, we have focused on fragment no. 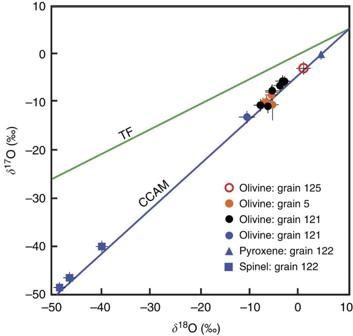125 where shock is most evident and could be studied with minimal sample loss. Figure 1: Oxygen isotope composition. A plot of oxygen three-isotope composition27to discriminate terrestrial (TF=terrestrial fractionation) and extraterrestrial (CCAM=carbonaceous chondrite anhydrous minerals) sources. The plot displays data for olivine from grain 125 (red open circle) with minerals from grains nos: 5 (orange solid symbols), 121 (black and blue solid symbols) and 122 (blue solid symbols) where the symbols correspond to pyroxene (triangles), olivine (circles) and spinel (squares) in the Khatyrka meteorite. All data are ion microprobe measurements made with the Cameca ims-7f geo. The error bars are 2σ. The plotted compositional indices,δ18OVSMOWandδ17OVSMOW(where VSMOW is Vienna Standard Mean Ocean Water), are the difference in18O/16O and17O/16O ratios, respectively, compared with the ratios in VSMOW, expressed in parts per thousand. Terrestrial minerals fall along the TF line (green line) with a slope of∼0.5; the oxygen isotope compositions measured for our samples lie along the line corresponding to anhydrous minerals in the CO or CV CC (blue line) with a slope of∼1. Figure 1: Oxygen isotope composition. A plot of oxygen three-isotope composition [27] to discriminate terrestrial (TF=terrestrial fractionation) and extraterrestrial (CCAM=carbonaceous chondrite anhydrous minerals) sources. The plot displays data for olivine from grain 125 (red open circle) with minerals from grains nos: 5 (orange solid symbols), 121 (black and blue solid symbols) and 122 (blue solid symbols) where the symbols correspond to pyroxene (triangles), olivine (circles) and spinel (squares) in the Khatyrka meteorite. All data are ion microprobe measurements made with the Cameca ims-7f geo. The error bars are 2 σ . The plotted compositional indices, δ 18 O VSMOW and δ 17 O VSMOW (where VSMOW is Vienna Standard Mean Ocean Water), are the difference in 18 O/ 16 O and 17 O/ 16 O ratios, respectively, compared with the ratios in VSMOW, expressed in parts per thousand. 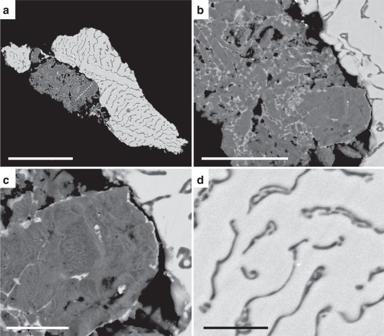Terrestrial minerals fall along the TF line (green line) with a slope of ∼ 0.5; the oxygen isotope compositions measured for our samples lie along the line corresponding to anhydrous minerals in the CO or CV CC (blue line) with a slope of ∼ 1. Figure 2: SEM backscattered electron images of sample no. 125. (a) An overall view of the sample showing the oval-shaped aggregate of silicates and oxides bordered by an intergrowth of nearly pure metallic Al (thin grey wavy) in khatyrkite, CuAl2(the brighter portions comprising most of the metallic grains); the two CuAl2grains are in the same crystallographic orientation, based on electron backscattered diffraction (EBSD), and a re-polishing of the sample demonstrated that the two pieces are physically continuous; a FIB section was taken from the area indicated with the white dotted line; (b) close-up of the sample showing the fragmented nature of the silicate assemblage; (c) close-up of the silicate portion of the grain showing olivine with spinel-filled veins (thin light stripes) and the magnetite rim adjacent to the CuAl2metal; (d) khatyrkite (CuAl2) with wavy eutectic structure of nearly pure aluminium similar to that reported by Zimmermanet al.16Scale bars, 50 μm (a); and 5 μm (b–d). Full size image Figure 2: SEM backscattered electron images of sample no. 125. ( a ) An overall view of the sample showing the oval-shaped aggregate of silicates and oxides bordered by an intergrowth of nearly pure metallic Al (thin grey wavy) in khatyrkite, CuAl 2 (the brighter portions comprising most of the metallic grains); the two CuAl 2 grains are in the same crystallographic orientation, based on electron backscattered diffraction (EBSD), and a re-polishing of the sample demonstrated that the two pieces are physically continuous; a FIB section was taken from the area indicated with the white dotted line; ( b ) close-up of the sample showing the fragmented nature of the silicate assemblage; ( c ) close-up of the silicate portion of the grain showing olivine with spinel-filled veins (thin light stripes) and the magnetite rim adjacent to the CuAl 2 metal; ( d ) khatyrkite (CuAl 2 ) with wavy eutectic structure of nearly pure aluminium similar to that reported by Zimmerman et al. [16] Scale bars, 50 μm ( a ); and 5 μm ( b – d ). Full size image Figure 3: Comparison of shocked and unshocked textures. Backscattered electron images of the shocked silicate textures in grain no. 125 ( a ) compared with the unshocked textures in Khatyrka matrix ( b ) from grain no. 5. Note that the ‘olivine’ grains in the left image have the same sizes and distinctive shapes as those in unshocked Khatyrka matrix, showing that the matrix was the precursor for the shocked silicates. Al, metallic aluminium; Kh, khatyrkite; Ol, olivine; ‘Ol’, shocked olivine grains, now consisting of ahrensite+forsterite+glass+spinels. Scale bars, 10 μm. Full size image Evidence of shock pressures that exceeded 5 GPa The silicates and oxides in sample no. 125 provide strong evidence of shock pressures that exceeded 5 GPa. In particular, we report here the presence of two high-pressure mineral phases: ahrensite, observed for the first time in a CV3 CC, and a new oxide spinelloid. The olivine grains of sample 125 are laced by a network of fine veins ( Fig. 2c ), each of which, under transmission electron microscopy (TEM) magnification, resembles a ‘ladder’ made up of alternating ‘rungs’ of ahrensite and of an amorphous SiO 2 -rich phase ( Figs 4 and 5 ), similar to phases found in the Umbarger L6 chondrite [11] . Ahrensite can only form at pressures exceeding 5 GPa (ref. 12 ). The ladders, the olivine hosts to the ladders and other silicates are cut by a network of fractures ( Fig. 2b,c ). These fractures, and interstices at triple junctions between olivine grains, are filled by nanometre-scale subhedral spinel crystals (bright in the scanning electron microscopy (SEM) backscattered electron images of Fig. 2b,c ). Among these is a phase ( Fig. 6a,c ) with composition Fe 3− x Si x O 4 (with x ≈0.4—TEM–energy dispersive spectrometry (TEM–EDS) data) and the orthorhombic structure reported for spinelloid V [13] . The occurrence of the spinelloid in this set of veins/fractures implies pressures of 3–8 GPa (ref. 13 ). See also Figs 7 and 8 for evidence of other new mineral phases (discussed below). 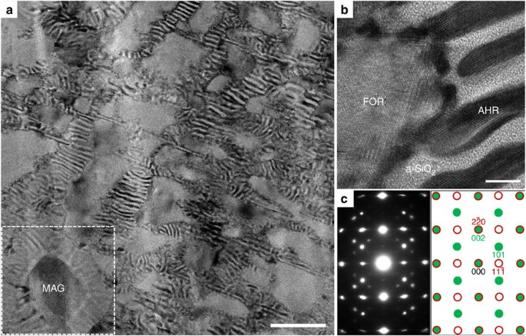Figure 4: Ladder-like veins. (a) TEM image from the FIB sample taken from a portion of the grain reported inFig. 2ashowing ladder-like veins (lamellar eutectic structure) of ahrensite (AHR) and an amorphous SiO2-rich phase (a-SiO2,Fig. 4b). In lower left part of the figure is an equant magnetite grain (MAG) surrounded by ladder veins (the white dotted box is shown enlarged inFig. 5). (b) Close-up of ladder showing olivine (FOR) and ahrensite (AHR) regions whose electron diffraction patterns (along [010] and [112] zone axes, respectively) were obtained and superposed inc, showing that the two minerals exhibit a crystallographic alignment (green and empty circles refer to forsterite and ahrensite, respectively). Similar alignments were found throughout regions ina. Scale bars, 200 nm (a) and 5 nm (b). Figure 4: Ladder-like veins. ( a ) TEM image from the FIB sample taken from a portion of the grain reported in Fig. 2a showing ladder-like veins (lamellar eutectic structure) of ahrensite (AHR) and an amorphous SiO 2 -rich phase (a-SiO 2 , Fig. 4b ). In lower left part of the figure is an equant magnetite grain (MAG) surrounded by ladder veins (the white dotted box is shown enlarged in Fig. 5 ). ( b ) Close-up of ladder showing olivine (FOR) and ahrensite (AHR) regions whose electron diffraction patterns (along [010] and [112] zone axes, respectively) were obtained and superposed in c , showing that the two minerals exhibit a crystallographic alignment (green and empty circles refer to forsterite and ahrensite, respectively). Similar alignments were found throughout regions in a . Scale bars, 200 nm ( a ) and 5 nm ( b ). 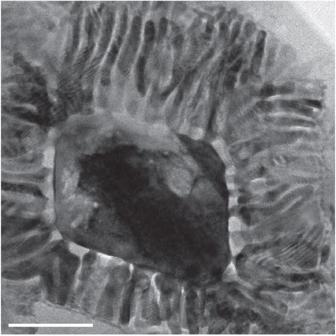Figure 5: Magnetite grain surrounded by ladder veins. The observed texture suggests that the ladders could have formed by a reaction between forsterite and magnetite, producing a melt with the bulk composition of the ladders. Scale bar, 100 nm. Full size image Figure 5: Magnetite grain surrounded by ladder veins. The observed texture suggests that the ladders could have formed by a reaction between forsterite and magnetite, producing a melt with the bulk composition of the ladders. Scale bar, 100 nm. 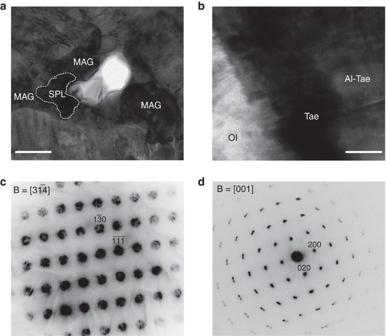Figure 6: TEM images of oxide and metallic phases. (a) Spinelloid V (SPL) with composition Fe3−xSixO4(withx≈0.4—TEM-EDS data) coexisting with magnetite (MAG) in fracture (bright white spot is a hole); scale bar, 200 nm; (b) Al–Cu-bearing taenite (Al-Tae) associated with taenite (Tae) and olivine (Ol); scale bar, 50 nm. TEM-EDS data give Fe44Ni26Al18Cu12, Fe51Ni36Cu13and (Mg1.95Fe0.05)SiO4; (c) convergent beam electron diffraction pattern along the [] zone axis of the spinelloid V shown ina; (d) electron diffraction pattern of Al–Cu-bearing taenite shown inbdown the [001] zone axis; the cubic cell parameter measured is 3.67(±1) Å. Full size image Figure 6: TEM images of oxide and metallic phases. ( a ) Spinelloid V (SPL) with composition Fe 3− x Si x O 4 (with x ≈0.4—TEM-EDS data) coexisting with magnetite (MAG) in fracture (bright white spot is a hole); scale bar, 200 nm; ( b ) Al–Cu-bearing taenite (Al-Tae) associated with taenite (Tae) and olivine (Ol); scale bar, 50 nm. TEM-EDS data give Fe 44 Ni 26 Al 18 Cu 12 , Fe 51 Ni 36 Cu 13 and (Mg 1.95 Fe 0.05 )SiO 4 ; ( c ) convergent beam electron diffraction pattern along the [ ] zone axis of the spinelloid V shown in a ; ( d ) electron diffraction pattern of Al–Cu-bearing taenite shown in b down the [001] zone axis; the cubic cell parameter measured is 3.67(±1) Å. 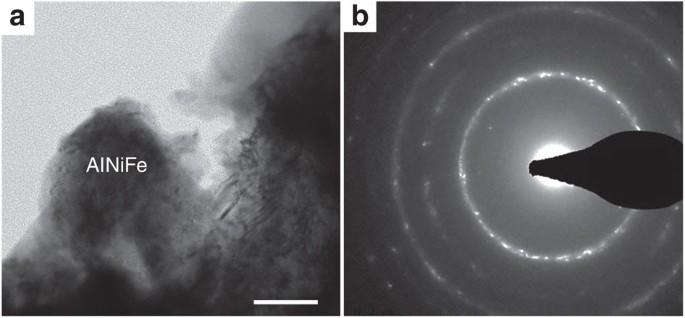Figure 7: A potential new mineral. (a) An unnamed AlNiFe phase with composition Al0.38Ni0.32Fe0.30(WDS data), whose diffraction pattern (b) was indexed according to a bcc structure witha=3.02(±1) Å. Scale bar, 50 nm. Full size image Figure 7: A potential new mineral. ( a ) An unnamed AlNiFe phase with composition Al 0.38 Ni 0.32 Fe 0.30 (WDS data), whose diffraction pattern ( b ) was indexed according to a bcc structure with a =3.02(±1) Å. Scale bar, 50 nm. 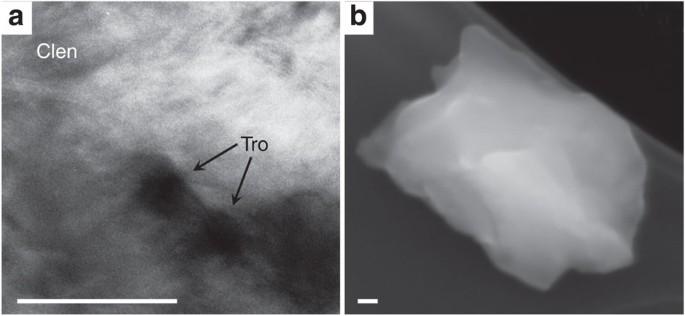Figure 8: Al- and Cu-bearing sulphides. (a) Cu-bearing troilite (Tro) with composition (Fe0.47Ni0.28Cu0.25)S (TEM-EDS data) associated with clinoenstatite (Clen) with composition (Mg1.80Fe0.20)Si2O6(TEM-EDS data); (b) Al-bearing iron sulphide with composition (Fe0.84Al0.04)S1.12(SEM-EDS data). Scale bar, 50 nm. Full size image Figure 8: Al- and Cu-bearing sulphides. ( a ) Cu-bearing troilite (Tro) with composition (Fe 0.47 Ni 0.28 Cu 0.25 )S (TEM-EDS data) associated with clinoenstatite (Clen) with composition (Mg 1.80 Fe 0.20 )Si 2 O 6 (TEM-EDS data); ( b ) Al-bearing iron sulphide with composition (Fe 0.84 Al 0.04 )S 1.12 (SEM-EDS data). Scale bar, 50 nm. Full size image Evidence of temperatures reaching about 1,200 °C The ladder veins cutting the olivine provide evidence that portions of the sample reached a temperature of at least 1,200 °C. We plot the compositions of the Si–Fe–Mg phases in Fig. 9 . Although most of the Fe-rich spinels in the spinel-filled veins plot at the Fe corner of Fig. 9 , some contain silicon, including the spinelloid. On average, the composition of the other low Ni spinels in the fractures is (Mg 0.94 Fe 0.78 Al 1.01 Ni 0.27 )O 4 . Neglecting Al and Ni, this composition projects onto the Fe–Mg–Si diagram in Fig. 9 at the inverted triangle. 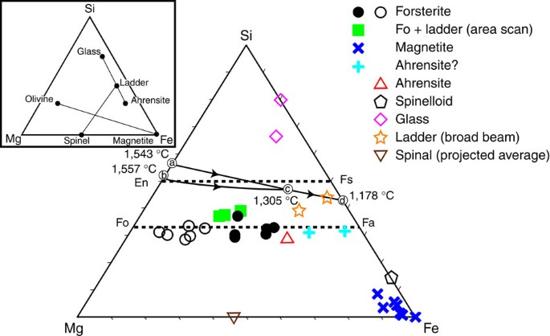Figure 9: Compositions of phases plotted in terms of normalized Si–Fe–Mg. Results (in atomic %) are based on SEM-EDS (closed symbols) and TEM-EDS (open symbols) measurements. Projections of the cotectic and reaction paths on the low pressure liquidus for the system MgO–FeO–SiO2(ref.14) are shown by lines with arrows. Between 1,543 and 1,305 °C is the silica-pyroxene cotectic (a–c); between 1,557 and 1,305 °C is the pyroxene-olivine reaction path (b–c); and between 1,305 and 1,178 °C is the silica-olivine cotectic (c–d). Along the forsterite (Fo)–fayalite (Fa) join, the analyses range from Fo89(TEM) to Fo11(SEM). (En, enstatite; Fs, ferrosilite). The bulk compositions of the ladders (obtained by broad beam TEM-EDS) are shown as open stars. They lie off the Fo–Fa join towards Si, and are close to the olivine-silica cotectic. Averaged TEM-EDS analyses (obtained using a beam size of 2 nm) are shown as open diamonds for the silica rungs of the ladders, and as open triangle for the ahrensite rungs. The SEM-EDS analyses plotted as plus signs may also be ahrensite in that they are more Fe rich than the identified ahrensite. The three filled squares are analyses from SEM-EDS scans over relatively large areas of olivine grains. These include the Fe-rich veins referred to as ladders. These analyses lie between the TEM-EDS forsterite analyses (open circles) and the TEM-EDS broad beam ladder analyses (open stars). This is consistent with the compositions determined by the SEM X-ray area scans to lie along a mixing line between the ladder compositions and forsterite. The SEM-EDS area scans show the relative enrichment of Si in the composite grain due to the presence of the silica phase in the ladders. The inset illustrates reactions discussed in the text: the crossing tie lines show the reaction olivine+magnetite=ladder+spinel. Because the spinel also contains Ni and Al, the reactants must include phases with Ni and Al (or a phase that contains both, such as shown inFigs 6band7a). Also shown are silica and ahrensite that formed from rapidly cooled liquid with the composition of the ladders (open stars). Figure 9: Compositions of phases plotted in terms of normalized Si–Fe–Mg. Results (in atomic %) are based on SEM-EDS (closed symbols) and TEM-EDS (open symbols) measurements. Projections of the cotectic and reaction paths on the low pressure liquidus for the system MgO–FeO–SiO 2 (ref. 14 ) are shown by lines with arrows. Between 1,543 and 1,305 °C is the silica-pyroxene cotectic ( a – c ); between 1,557 and 1,305 °C is the pyroxene-olivine reaction path ( b – c ); and between 1,305 and 1,178 °C is the silica-olivine cotectic ( c – d ). Along the forsterite (Fo)–fayalite (Fa) join, the analyses range from Fo 89 (TEM) to Fo 11 (SEM). (En, enstatite; Fs, ferrosilite). The bulk compositions of the ladders (obtained by broad beam TEM-EDS) are shown as open stars. They lie off the Fo–Fa join towards Si, and are close to the olivine-silica cotectic. Averaged TEM-EDS analyses (obtained using a beam size of 2 nm) are shown as open diamonds for the silica rungs of the ladders, and as open triangle for the ahrensite rungs. The SEM-EDS analyses plotted as plus signs may also be ahrensite in that they are more Fe rich than the identified ahrensite. The three filled squares are analyses from SEM-EDS scans over relatively large areas of olivine grains. These include the Fe-rich veins referred to as ladders. These analyses lie between the TEM-EDS forsterite analyses (open circles) and the TEM-EDS broad beam ladder analyses (open stars). This is consistent with the compositions determined by the SEM X-ray area scans to lie along a mixing line between the ladder compositions and forsterite. The SEM-EDS area scans show the relative enrichment of Si in the composite grain due to the presence of the silica phase in the ladders. The inset illustrates reactions discussed in the text: the crossing tie lines show the reaction olivine+magnetite=ladder+spinel. Because the spinel also contains Ni and Al, the reactants must include phases with Ni and Al (or a phase that contains both, such as shown in Figs 6b and 7a ). Also shown are silica and ahrensite that formed from rapidly cooled liquid with the composition of the ladders (open stars). Full size image The cotectic and reaction paths on the liquidus in the MgO–FeO–SiO 2 system [14] are shown by lines with arrows in Fig. 9 ; we here interpret our results in terms of the low-pressure olivine-silica cotectic (there are no high-pressure experimental data on this system), from the ternary peritectic (c, Fig. 9 ) at 1,305 °C to the binary eutectic (d, Fig. 9 ) at 1,178 °C. The bulk composition of the ladders lies near the Fe-rich olivine-silica cotectic (c,d in Fig. 9 ), which is consistent with an interpretation that the ladders formed from a melt at about 1,200 °C. Following formation of the melts with the bulk composition of the ladders, the silica-rich phase and the ahrensite formed from a liquid with composition on the cotectic, with the compositions of the combined phases adding up to the bulk composition of the ladders. The enrichment of Si in the ladders compared with the Si content of olivine and the much higher Fe/Mg of the ladders than the host forsterite (Fo 80–85 ) imply an open system to produce a change in composition from forsterite to ahrensite+SiO 2 . The texture of the ladders between the 200-nm magnetite grain and forsterite ( Figs 4a and 5 ) suggests that the ladders could have formed by a reaction between forsterite and magnetite, producing a melt with the bulk composition of the ladders; the Mg produced in this reaction may be in the spinels (inverted triangle in Fig. 9 ) that precipitated in the fractures. In Fig. 9 , considering only the Mg, Fe and Si components, a reaction is implied involving forsterite+magnetite as reactants and the ladders+spinel as products (see inset in Fig. 9 ). Evidence of rapid cooling The composition of the whole Al+CuAl 2 grain that partially encloses the silicate assemblage ( Fig. 2a ) is close to the peritectic (at about 600 °C) in the Al–Cu system (30% Cu and 70% Al [15] ), consistent with the metal solidifying late during the cooling. The grains exhibit a wavy eutectic structure ( Fig. 2a,d ) composed of nearly stoichiometric khatyrkite (CuAl 2 , containing 0.8% Fe) and Al metal (containing 1% Cu). This texture is known to occur as a result of rapid cooling ( ∼ 10 2 –10 3 °C s −1 ) of liquids in the Al–Cu system [16] , [17] , [18] . The lamellar eutectic texture of the ladder areas is also typical for a rapidly cooled composition beginning from a temperature near the olivine-silica cotectic in the MgO–FeO–SiO 2 system ( Fig. 9 ). Further evidence of rapid cooling is the presence of the amorphous high silica phase. The extreme difference in Mg number between the forsterite (Fo 80 ) and the average ladder (Fo 20 ) shows that the liquid was not in equilibrium with the host forsterite, despite the extremely small size of our samples. The absence of any reaction between the ladders and the host, considering the ease of diffusive equilibration of olivine, is a further indication of a very rapid cooling. The Cu–Al grain cuts across the trends of the spinel-filled fractures and veins ( Fig. 2b,c ) and of the ladders; therefore, it was the last portion of sample 125 to solidify. The thin rim of magnetite on the olivine adjacent to the CuAl 2 composite grain ( Fig. 2b ) may be a vein wall, like the other thin spinel-filled veins. The lack of reaction between the highly reduced metallic Al-bearing metal of the metal nodule and the magnetite between the olivine and the Cu–Al metal strongly suggests that the sample cooled too fast, and to too low of a temperature, for diffusion between the incompatible phases to occur. Finally, evidence for rapid cooling can be observed by comparing the textures in the Khatyrka sample with those found in controlled laboratory rapid-cooling experiments [19] . (Although sample no. 125 does not include icosahedrite, here we consider the collection of phases observed in the various grains from Khatyrka.) In the ternary diagram for Al–Cu–Fe, there is a small range of liquid compositions where icosahedrite is on the liquidus between 850 and 700 °C (see Figs 1 and 2 in Zhang and Lück [20] ). This region is reached through a liquid line of descent from higher temperatures. During crystallization of icosahedrite from a liquid, a ternary peritectic with the phase omega (Cu 2 FeAl 7 ) is reached and the icosahedrite reacts out of the system. With further cooling, cupalite crystallizes together with omega along a cotectic until a ternary eutectic is reached where khatyrkite joins cupalite and omega. The composition of this residual liquid is very close to the composition of the binary peritectic with cupalite and khatyrkite; subsolidus phase diagrams for these compositions show that omega is the stable phase with khatyrkite and cupalite [19] , [20] . However, in Khatyrka, the samples do not have the phase omega. Zhang and Lück [21] point out that omega does not appear in rapidly cooled liquid compositions where icosahedrite is on the liquidus; instead, those compositions end up with an assemblage of khatyrkite-cupalite-icosahedrite-β (where β is AlCuFe solid solution); this assemblage is observed in Khatyrka, with icosahedrite and β remaining as unreacted phases in an assemblage containing cupalite and khatyrkite (see Fig. 2 in Bindi et al. [1] ). Al- and Cu-bearing FeNi metals The presence of Al- and Cu-bearing FeNi metals is a strong evidence that FeNi and the Al–Cu-bearing metals coexisted during the impact shock. A critical finding is the discovery of two new minerals, Al–Cu-bearing taenite (Al-Tae) associated with taenite (Tae) and olivine (Ol) ( Fig. 6b,d ) and an unnamed AlNiFe phase with composition Al 0.38 Ni 0.32 Fe 0.30 ( Fig. 7 ). In addition, we have found a Cu-bearing troilite ( Fig. 8a ) and an Al-bearing iron sulphide ( Fig. 8b ). The cubic cell parameter measured for taenite is 3.67(±1) Å, slightly larger than that reported for pure taenite [22] (that is, 3.58 Å), in agreement with the incorporation of the larger Al ion [23] in the structure. The diffraction pattern of Al 0.38 Ni 0.32 Fe 0.30 was indexed according to a bcc structure with a =3.02(±1) Å, which corresponds to the A2 structure in the Al–Ni–Fe system [24] . The presence of khatyrkite, cupalite and icosahedrite with the Al–Cu-bearing taenite in the CV3 CC suggests that Al- and Cu-bearing FeNi metals were transported during the shock event without any significant oxidation reaction, which is plausible if the shock event occurred in contact with the highly reducing solar nebula gas. Studies by Rubin [25] identified examples of ordinary chondrites containing Cu-bearing FeNi grains that underwent impacts and suggested that the impacts led to shock-generated melting and the extraction of the Cu into metallic droplets. Now we have observed in Khatyrka that FeNi can host Al and Cu, both separately and together. The Al- and Cu-bearing FeNi phases might have been the initial source of the CuAl metals (khatyrkite, cupalite and icosahedrite), thus explaining how the lithophilic Al and chalcophylic Cu became associated. Alternatively, the Al–Cu metals may have had a pre-accretion nebular origin and the Al- and Cu-bearing taenite observed in the sample formed by shock-induced reaction of the Cu–Al melt and taenite. We discuss both possibilities below. One hypothesis for explaining the properties of Khatyrka described above is that the shock we have documented locally generated the heat and pressure necessary to extract Al and Cu from the FeNi metals and to initiate the local melting of metals and silicate; the Al and Cu would then be dissolved in a silicate melt from which the Al–Cu–Fe alloys precipitated, along with forsterite and diopside (see Fig. 1 in Bindi et al. [5] ). The local, transient ultra-high pressures led to the nucleation and growth of ahrensite and spinelloid V. Icosahedrite could have grown from melted metals, and stishovite could have grown around it while the pressure was still high, thus explaining the stishovite grains with icosahedrite inclusions found in the original museum sample [5] . The alternate hypothesis is that the Cu–Al metals formed in some nebular process before the impact that formed the silicate ladders and that the impact resulted in the remelting, rapid cooling and solidification of the CuAl metals. This hypothesis has the advantages that it can naturally account for the icosahedrite inclusions in stishovite and that it can explain why CuAl metal grains are found in some other Khatyrka samples—for example, grain nos: 5 and 121—that show no evidence of shock [7] . In either model, the sequence of events that formed Khatyrka’s metal must have occurred in contact with the reducing solar nebula gas. If the magnetite present in our sample is indicative of oxidizing conditions during the shock event, then that process must have been so rapid that there was no equilibration of oxygen with the metals. The properties described above cannot plausibly be explained as being due to terrestrial atmospheric entry and impact. Atmospheric entry is far too oxidizing and the pressure does not reach the values indicated by ahrensite and spinelloid V. The formation of ahrensite and stishovite requires very high pressures, not just high temperatures, which could only occur in hypervelocity impacts that would leave sizeable craters. On the basis of the sediments hosting the grains, the impact likely occurred <10 Ka (ref. 7 ), and no evidence of a significant crater formed since has been found in our studies of the region. By contrast, taking into account the presence of Cu in moderating the fugacity requirements to form metallic Al, the reducing conditions needed to make the metal are consistent with those inferred to exist in the presolar nebula at 4.5 Ga (ref. 26 ). According to our first hypothesis, the Cu and Al are extracted from the FeNi lattice as a result of the impact; according to the second, CuAl metals already existed before impact and the Cu and Al subsequently entered the FeNi. Either way, this exchange of metallic Al and Cu can only be plausibly imagined to occur in space under solar nebular conditions, and not during terrestrial entry and impact. Both hypotheses leave open the very challenging question of how the metallic Al- and Cu-bearing phases, whether AlCu-bearing FeNi for the first hypothesis or AlCu alloy for the second hypothesis, formed in the first place given that Al and Cu have two profoundly different cosmochemical properties and normally condense under very different conditions. What we have established is that, in either explanation, impact shock in space that occurred billions of years ago played a key role in the formation of icosahedrite and other Al–Cu-bearing alloys, as well as the combination of other unusual phases observed in Khatyrka, including several phases never seen before in a CV3 CC and some never seen before in any natural material. Experiments are now underway to study the stability of icosahedrite at high pressures and temperatures, and to recreate in the laboratory the high-pressure shock-melting conditions that could have triggered the extraction of Al and Cu from FeNi phases. These studies may enable us to test and distinguish our hypotheses. Sample characterization techniques The samples studied here (nos: 125 and 126 recovered from the expedition in the Koryak Mts. [6] , [7] ) were investigated by means of EDS, SEM, focused ion beam (FIB), WDS (wavelength dispersive spectrometry) and TEM techniques. An olivine fragment from sample 125 was selected for the SIMS (secondary ion mass spectrometry) O-isotope studies. Scanning electron microscopy Grains nos: 125 and 126 were first investigated with a SEM. The instrument used was a FEI Quanta 200 FEG Environmental-SEM equipped with an Oxford INCA Synergy 450 energy-dispersive X-ray microanalysis system, operated at 15 and 5 kV accelerating voltage, 140 pA probe current, 2,000 c.p.s. as average count rate on the whole spectrum and a counting time of 60 s. Samples were sputter coated with a 5-nm-thick carbon film. The lower voltages were used to minimize secondary radiation from adjacent phases. Standards for the metals and olivine were forsterite (Mg, Si) and synthetic icosahedrite (Al, Cu, Fe). Electron microprobe We carried out WDS electron microprobe analyses on an AlNiFe grain (about 5 μm in size, larger than the one in Fig. 7a and showing an almost tabular morphology) using a JEOL JXA-8600 electron microprobe operating at an accelerating voltage of 15 kV, beam current of 20 nA and a beam diameter of 1 μm. Variable counting times were used: 30 s for Al, Ni and Fe, and 60 s for the minor elements Mg, Si, Cr, P, Co, Cu, Cl, Ca, Zn and S. Replicate analyses of synthetic Al 53 Ni 42 Fe 5 were used to check accuracy and precision. The crystal fragment was found to be homogeneous within analytical error. The standards used were: metal-Al (Al), synthetic Ni 3 P (Ni, P), synthetic FeS (Fe), metal-Mg (Mg), metal-Si (Si), metal-Cr (Cr), metal-Co (Co), metal-Cu (Cu), synthetic CaCl 2 (Ca, Cl) and synthetic ZnS (Zn, S). FIB and TEM In preparation for the study with TEM, a thin lamella cross-section from sample no. 125 was collected using the FIB technique. The sample was prepared using a standard process for deep trench milling and lift out in the FIB/SEM Hitachi NB5000. Final milling was performed using a fine 5 kV Ga + beam of 120 nA for cleaning and amorphous removal from the front and back side of the lamella. The thickness of the final lamella is <80 nm. The subsequent TEM study was done using a Philips CM200-FEG TEM (operating at 200 KeV) operated using the standard high-resolution imaging and micro/nano diffraction mode. Another JEOL JEM 2010 (operating at 200 kV with an ultra-high resolution pole piece, and a point-to-point resolution close to 1.9 Å) was also used. The FIB section was studied only using the Philips CM200-FEG TEM, whereas a powder from sample no. 126 was studied using both TEMs. The powder from sample no. 126 was placed on an Au mesh TEM grid (300 mesh, 3 mm in diameter) that was previously covered by a thin carbon layer (support film). EDS data were obtained using Evex NanoAnalysis System IV attached to the Philips CM200-FEG TEM. A small electron probe of 20–100 nm was used with a count rate of 100–300 c.p.s. using an average collection time of 180 s. The quantitative analyses were done at 200 kV and are based on using pure elements and the NIST 2063a standard sample as a reference under the identical TEM operating conditions. Secondary ion mass spectrometry Oxygen isotopic compositions, to discriminate terrestrial and extra-terrestrial minerals [27] , of a large olivine grain were obtained using the Cameca ims-7f geo ion microprobe ( Fig. 1 ). The measurements were made with a relatively large ( ∼ 15 μm), intense (0.2 nA) primary ion beam and resulted in relatively precise measurements ( ∼ ±2–2.5‰ for both 17 O and 18 O, 2 σ ) of the isotopic compositions in a large olivine grain. Standards used for this analysis are San Carlos olivine, Eagle Station olivine and Burma spinel. Secondary ions were collected by peak jumping into either a Faraday cup ( 16 O − ) or electron multiplier ( 17 O − and 18 O − ) at a mass resolving power of ∼ 6,500, easily resolving the 16 OH − interference on 17 O − . How to cite this article: Hollister, L. S. et al. Impact-induced shock and the formation of natural quasicrystals in the early solar system. Nat. Commun. 5:4040 doi: 10.1038/ncomms5040 (2014).